Two-dimensional superconductivity at the interface of a Bi2Te3/FeTe heterostructure The realization of superconductivity at the interface between a topological insulator and an iron-chalcogenide compound is highly attractive for exploring several recent theoretical predictions involving these two new classes of materials. Here we report transport measurements on a Bi 2 Te 3 /FeTe heterostructure fabricated via van der Waals epitaxy, which demonstrate superconductivity at the interface, which is induced by the Bi 2 Te 3 epilayer with thickness even down to one quintuple layer, though there is no clear-cut evidence that the observed superconductivity is induced by the topological surface states. The two-dimensional nature of the observed superconductivity with the highest transition temperature around 12 K was verified by the existence of a Berezinsky–Kosterlitz–Thouless transition and the diverging ratio of in-plane to out-plane upper critical field on approaching the superconducting transition temperature. With the combination of interface superconductivity and Dirac surface states of Bi 2 Te 3 , the heterostructure studied in this work provides a novel platform for realizing Majorana fermions. The emergent realization of superconductivity at the interfaces between transition metal oxides has attracted growing attention in recent years [1] . Typical transition metal oxide interfaces reported so far include LaAlO 3 /SrTiO 3 (LAO/STO), LaTiO 3 /SrTiO 3 , La 2 CuO 4 /La 2− x Sr x CuO 4 and Ba 1− x Nd x CuO 2 /CaCuO 2 (refs 2 , 3 , 4 , 5 , 6 , 7 ). Interface superconductivity between chalcogenides such as PbTe/PbSe and PbSe/PbS has also been reported [8] . Recently, the discovery of superconductivity in layered iron-based materials has steered the high-transition-temperature ( T c ) superconductors to an iron age. These so-called iron-based superconductors (Fe-SC) are the focus of contemporary research due to their high upper critical fields, large critical current densities and unconventional pairing symmetries. Among them, the 11-type iron-chalcogenide Fe-SCs have the simplest chemical composition and a relatively simple crystalline structure [9] , [10] , [11] . Since the discovery of Fe-SC in 2007, another novel state of quantum matter, the topological insulator (TI), has become an important topic in condensed matter physics [12] , [13] . The robust topological surface states are topologically protected against time-reversal-invariant perturbations. More interestingly, inducing s -wave superconductivity on the surface state of a TI results in a p -wave superconductor that hosts Majorana fermions in its vortex cores [12] , [13] . Motivated by the prospect of creating Majorana fermions, which are non-Abelian particles and have potential applications in quantum computations [14] , several attempts have been made to induce superconductivity on TI surfaces using bulk superconductors [15] , [16] , [17] , [18] . In this work, we find that interface superconductivity is induced when a thin film of TI, Bi 2 Te 3, is grown on a non-superconducting FeTe thin film. We show that the resulting superconductivity possesses the characteristics of Fe-SCs with the highest T c of ~\n12 K. The superconductivity exhibits two-dimensional (2D) nature by showing the evidence of a Berezinsky–Kosterlitz–Thouless (BKT) transition and the diverging ratio of in-plane to out-plane upper critical field on approaching T c . Its superconducting thickness is estimated to be ~\n7.0±1.1 nm, based on the measured upper critical fields. This work provides the first example of interface superconductivity between a TI and iron chalcogenide. Due to the possible unconventional pairing symmetry of Fe-SC [19] , the Bi 2 Te 3 /FeTe heterostructures also provide new platforms for studying the interplay between unconventional superconductors and TI surface states as well as for creating Majorana fermions. Structural properties of the heterostructure Bi 2 Te 3 is one of the simplest three-dimensional TIs, whose surface states consist of a single Dirac cone at the Γ point [20] . Its unit cell is formed by 3 quintuple layers (QLs), bonded by van der Waals (vdW) forces along the [0001] direction. Each QL contains two atomic sheets of Bi and three atomic sheets of Te, which are covalently bonded. The unit cell of tetragonal FeTe is composed of two Te–Fe–Te triple layers stacked along the [001] direction. Also, the neighbouring triple layers are bonded via vdW force. Attributed to the vdW bonding nature, even though Bi 2 Te 3 possesses a sixfold symmetry and FeTe is in a fourfold symmetry with respect to their c-axis directions, the heteroepitaxial growth can still proceed, resulting an atomically sharp interface via vdW expitaxy that allows defect-free epitaxial growth on a substrate possessing large lattice mismatch or distinct crystalline structure as compared with those of the epilayers [21] . 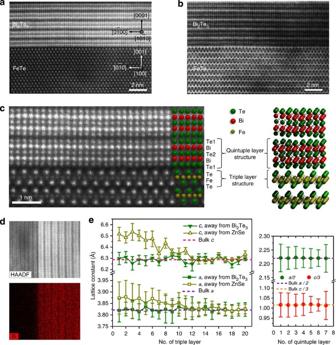Figure 1: Scanning transmission electron microscope micrographs of a Bi2Te3/FeTe heterostructure. (a) HADDF image. (b) Annular bright field image. (c) Higher-magnification HADDF image shows atomically sharp interface between Bi2Te3and FeTe. (d) Bi-EDS mapping across the interface. (e) Variation of the lattice parameters of FeTe (left) and Bi2Te3(right), extracted from their HAADF images, where the error bars specify the standard deviations of the measurements. Figure 1 displays the cross-section images of a Bi 2 Te 3 (7 QLs) /FeTe (140 nm) heterostructure taken by a spherical aberration-corrected scanning transmission electron microscope. Both high-angle annular dark field (HAADF) and annular bright field images, as shown in Fig. 1a,b , respectively, possess high contrast with significant sensitivity to the atomic number Z, and thus provide robust visibility of both light and heavy atoms. Figure 1c shows the high-magnification HAADF image of this heterostructure, in which one can see that the two layers are separated by a vdW gap and form their own lattices independently, confirming the growth is indeed via vdW epitaxy. Figure 1: Scanning transmission electron microscope micrographs of a Bi 2 Te 3 /FeTe heterostructure. ( a ) HADDF image. ( b ) Annular bright field image. ( c ) Higher-magnification HADDF image shows atomically sharp interface between Bi 2 Te 3 and FeTe. ( d ) Bi-EDS mapping across the interface. ( e ) Variation of the lattice parameters of FeTe (left) and Bi 2 Te 3 (right), extracted from their HAADF images, where the error bars specify the standard deviations of the measurements. Full size image Electrical and magneto-transport properties It is well-known that FeTe, as the parent compound of iron chalcogenides, does not exhibit superconductivity either at ambient pressure or under high hydrostatic pressure [22] , [23] , [24] , [25] , [26] . 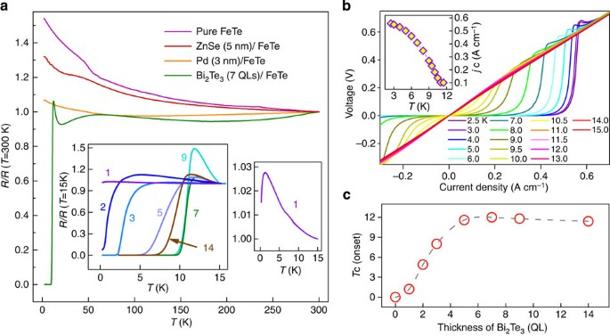Figure 2: Results of transport measurements. (a) Temperature-dependent resistanceR(T)/R(T=300 K) of pure FeTe, ZnSe/FeTe and Pd/FeTe films as well as a Bi2Te3(7 QLs)/FeTe heterostructure. The room temperature resistances of these samples are 16.1, 18.7, 5.0 and 22.5 Ω, respectively. The bottom left inset shows theR(T)/R(T=15 K) versus temperature of Bi2Te3/FeTe heterostructures with Bi2Te3thicknesses labelled in units of QL, while the bottom right inset is a finer scale plot for a Bi2Te3(1 QL)/FeTe heterostructure. (b) Current density-dependent voltage of the Bi2Te3(7 QLs)/FeTe heterostructure at different temperatures. The inset shows its temperature-dependent critical current density. (c)Tc(onset)versus the thickness of Bi2Te3thin film in units of QL. The dash line is a guide to the eyes. Figure 2a shows the resistance versus temperature R ( T ) curves for a pure 140-nm-thick FeTe film and a set of Bi 2 Te 3 /FeTe heterostructure samples with different thicknesses of Bi 2 Te 3 , while the thickness of the FeTe film is fixed at 140 nm. All these curves display a common drop around 50 K, which is attributed to the antiferromagnetic transition of FeTe [22] . The pure FeTe film does not show superconductivity down to 2 K. To further confirm the non-superconducting nature of the as-grown FeTe film, two additional FeTe (140 nm) samples were capped with Pd (3 nm) and ZnSe (5 nm), respectively, and in fact neither of their R ( T ) curves, which are displayed in Fig. 2a exhibit any superconductivity. However, the Bi 2 Te 3 /FeTe heterostructure samples with 3, 5, 7, 9 and 14 QLs of Bi 2 Te 3 undergo a transition into a state with zero resistance. The two heterostructure samples with 1 and 2 QLs of Bi 2 Te 3 also exhibit a resistance drop although the zero-resistance state has not been reached at the lowest temperature of 280 mK. Figure 2: Results of transport measurements. ( a ) Temperature-dependent resistance R ( T )/ R ( T =300 K) of pure FeTe, ZnSe/FeTe and Pd/FeTe films as well as a Bi 2 Te 3 (7 QLs)/FeTe heterostructure. The room temperature resistances of these samples are 16.1, 18.7, 5.0 and 22.5 Ω, respectively. The bottom left inset shows the R ( T )/ R ( T =15 K) versus temperature of Bi 2 Te 3 /FeTe heterostructures with Bi 2 Te 3 thicknesses labelled in units of QL, while the bottom right inset is a finer scale plot for a Bi 2 Te 3 (1 QL)/FeTe heterostructure. ( b ) Current density-dependent voltage of the Bi 2 Te 3 (7 QLs)/FeTe heterostructure at different temperatures. The inset shows its temperature-dependent critical current density. ( c ) T c(onset) versus the thickness of Bi 2 Te 3 thin film in units of QL. The dash line is a guide to the eyes. Full size image The electronic transport data of the heterostructure sample with 7 QLs of Bi 2 Te 3 (named as Sample A) obtained via standard four-probe method is displayed in Fig. 2b . One can see that the current density-dependent voltage V ( j ) of this sample shows a step-like critical current density profile at temperature below 11.0 K. This characteristic V ( j ) dependence together with the occurrence of a zero-resistance state provide unambiguous evidences for the existence of superconductivity in the Bi 2 Te 3 /FeTe heterostructure. The temperature-dependent critical current density ( j c ) (defined as the current density at the maximum derivative resistance) as shown in the inset of Fig. 2b enjoys a large magnitude of 10 −1 A cm −1 cm. 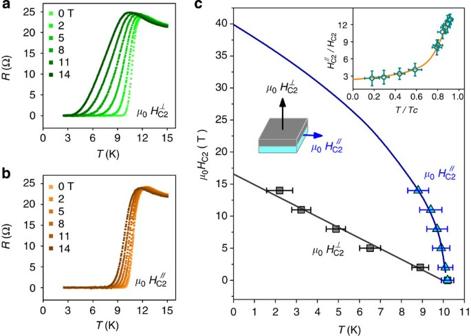Figure 3: Upper critical fields of Sample A. R(T) characteristics of Sample A measured under different magnetic fields in directions (a) perpendicular and (b) parallel to the interface. (c) Main panel: temperature-dependent upper critical fields in the directions parallel and perpendicular to the interface of Bi2Te3/FeTe heterostructure, where the error bars represent the range of the rounding region of the transition nearR=0. The curves are resulted from the fittings to the data based on the GL theory for 2D superconductors. Inset:as a function of reduced temperatureT/Tc, showing its diverging nature on approachingTc. Figure 3a,b , respectively, show that the superconductivity of this heterostructure sample cannot be fully destroyed by applying magnetic fields up to 14 T either vertical ( ) or parallel ( ) to the interface, which implies its upper critical field ( H C2 ) is quite large. The anomalous high j c and H C2 of the Bi 2 Te 3 /FeTe heterostructure sample (similar to those observed in Fe-SC) indicate that its superconductivity may be associated with the induced superconductivity of FeTe (to be discussed later). Furthermore, the superconducting transitions shown in Fig. 3a,b display a large anisotropy regarding the direction of the applied magnetic field since the transitions significantly broaden as increases, while such a broadening is much weaker as increases. Figure 3: Upper critical fields of Sample A. R ( T ) characteristics of Sample A measured under different magnetic fields in directions ( a ) perpendicular and ( b ) parallel to the interface. ( c ) Main panel: temperature-dependent upper critical fields in the directions parallel and perpendicular to the interface of Bi 2 Te 3 /FeTe heterostructure, where the error bars represent the range of the rounding region of the transition near R =0. The curves are resulted from the fittings to the data based on the GL theory for 2D superconductors. Inset: as a function of reduced temperature T / T c , showing its diverging nature on approaching T c . Full size image The important role of the Bi 2 Te 3 thin film for inducing the observed superconductivity in the Bi 2 Te 3 /FeTe heterostructure can be well supported by the results of transport measurements performed on a sample with a 140-nm-thick FeTe film capped with 7 QLs of Bi 2 Te 3 on half of the FeTe surface, named as Sample B (see Supplementary Fig. 1 ). The detailed characteristics of Sample B addressed in Supplementary Discussion demonstrate that the Bi 2 Te 3 thin film is indispensable for the observed superconductivity in the Bi 2 Te 3 /FeTe heterostructure. Evidences of 2D superconductivity It is worth to point out again the fact that all the Bi 2 Te 3 /FeTe heterostructures studied in this work exhibit superconductivity of which the thicknesses of their Bi 2 Te 3 thin films vary from 1 to 14 QLs (equivalent to ~\n1–14 nm), while pure Bi 2 Te 3 and FeTe films are not superconducting. This fact together with the indispensability of Bi 2 Te 3 in the observed superconductivity, as shown via Sample B, implies that the observed superconductivity originates from the interfaces of these heterostructures, suggesting that the source of the superconductivity may be confined to 2D. The confirmation of the 2D nature of the observed superconductivity can be obtained by testing whether the transport properties of the Bi 2 Te 3 /FeTe heterostructure possess a signature of a BKT transition that is well-known to be characterized by a BKT temperature ( T BKT ), below which a phase transition leading to a 2D topological order emerges [3] , [6] , [27] , [28] , [29] . 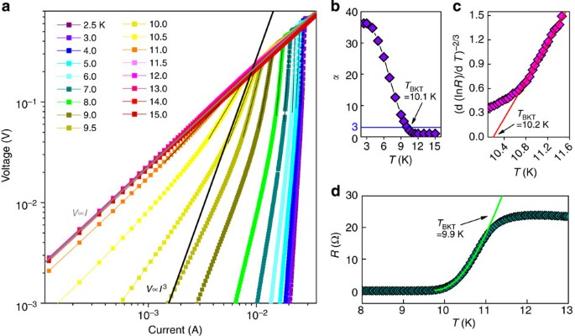Figure 4: BKT nature of Sample A. (a) Voltage-current density data plotted in a log–log scale. The short black lines are power-law fits of the data in the BKT transitions at different temperatures. The grey line corresponds to aV∝Ibehaviour while the black long line corresponds to aV∝I3behaviour. (b) Temperature dependence of the power-law exponentαdeduced from the power-law fits ina. The interception with the solid liney=3 gives aTBKT=10.1 K. (c)R(T) dependence plotted on a [dln(R)/dT]−2/3versusTscale. The solid line is the behaviour expected for a BKT transition withTBKT=10.2 K. (d)R(T) dependence with a fitting for a BKT behavior near the transition, yielding aTBKT=9.9 K. Figure 4a displays the I - V isotherms of Sample A on a log–log scale. The straight lines in this plot indicate the power-law behaviours, with the powers α equal to the slopes of the lines ( V ∝ I α ). Among them, the grey line with a slope of 1 coincides with the high-temperature isotherms (11.5~\n15.0 K), which indicates their ohmic characteristics ( V ∝ I ), while the long black line with a slope of 3 marks the initiation of a BKT transition ( V ∝ I 3 ). The short black lines are power-law fits to the data at different temperatures. It is worth pointing out that the standard BKT fitting is carried out for data points with current values less than the critical current values corresponding to different temperatures. However, when currents are smaller than some certain values, the system becomes ohmic due to finite-size effects (FSE) [30] . Thus, the fitting is usually applied to upper portion of the dataset, just below the critical currents. The slopes of the short black lines represent the powers α , which are plotted versus temperature in Fig. 4b . In this figure, the value of α approaches 3 at temperature of ~\n10.1 K, which is thus identified as T BKT , and increases rapidly for temperatures lower than 10.1 K. These observations are regarded as the hallmark of a BKT transition. On the other hand, at the temperature range just above T BKT , the temperature-dependent resistance is predicted to be in a form of R ( T ) ∝ R 0 exp[− b /( T − T BKT ) 1/2 ], where R 0 and b are material-specific parameters [3] , [6] , [27] , [28] , [29] . Both the plot of [d(ln R )/d T ] −2/3 versus T as shown in Fig. 4c and the best fit to the R ( T ) data using this form as shown in Fig. 4d agree well with the expected BKT behaviour near the transition, yielding T BKT equal to 10.2 and 9.9 K, respectively. These two resulting T BKT values are highly consistent with the value extracted from the power analysis—10.1 K. Our analysis thus provides strong evidences for a 2D nature of the observed superconductivity. Figure 4: BKT nature of Sample A. ( a ) Voltage-current density data plotted in a log–log scale. The short black lines are power-law fits of the data in the BKT transitions at different temperatures. The grey line corresponds to a V ∝ I behaviour while the black long line corresponds to a V ∝ I 3 behaviour. ( b ) Temperature dependence of the power-law exponent α deduced from the power-law fits in a . The interception with the solid line y =3 gives a T BKT =10.1 K. ( c ) R ( T ) dependence plotted on a [dln( R )/d T ] −2/3 versus T scale. The solid line is the behaviour expected for a BKT transition with T BKT =10.2 K. ( d ) R ( T ) dependence with a fitting for a BKT behavior near the transition, yielding a T BKT =9.9 K. Full size image Figure 3c shows the temperature-dependent upper critical field H C2 ( T ) for Sample A in directions parallel ( ) and perpendicular ( ) to the interface. The zero-resistance temperature (corresponding to the mid-point of the rounding region near R =0) is extracted from the R ( T ) characteristics under different and displayed in Fig. 3a,b . The corresponding H C2 ( T ) values derived from the zero-resistance temperatures were used to estimate the Ginzburg–Landau (GL) coherence length ξ GL and superconducting thickness d sc in our Bi 2 Te 3 (7 QLs)/FeTe heterostructure. It is noted that upper critical field for the parallel field direction follows the GL form of temperature-dependent behaviour for a 2D superconducting film, , where Φ 0 is the flux quantum and ξ GL (0) is the GL coherence length at T =0 K, and the resulting fitting curve is shown in Fig. 3c as well. In the perpendicular field direction, shows the expected linear T dependence, which follows the standard linearized GL theory for 2D superconductors, . The derived H C2 ( T ) values were used to plot the ratio versus reduced temperature T / T c (inset of Fig. 3c ) and it shows a diverging characteristic on approaching T c , characteristic for a 2D nature [31] . Using this temperature-dependent relationship, the mean value of ξ GL (0) can be calculated to be 5.2±1.7 nm. The mean value of superconducting thickness d sc is then estimated to be 7.0±1.1 nm using based on the extracted values and fittings. The fact that the zero-temperature critical field of our Bi 2 Te 3 /FeTe heterostructures is much larger than the fields used in taking the data for performing the fitting will certainly cause a substantial uncertainty in the estimations of both ξ GL and d sc . As their fitted values are quite close, one can still regard as a further confirmation for the 2D nature of the observed superconductivity, which is mainly demonstrated by the good match of the transport data with the BKT model and the diverging ratio of on approaching T c . It is worth pointing out that in parallel applied fields, the upper critical field (orbital limit for superconductivity) may be replaced by the Pauli limit for superconductivity. However, in the derivation of the coherence length the extrapolated orbital limit must be used, which agrees with our method of extrapolating the critical field line from our data at low fields close to the zero field critical temperature. In the following, we would perform the study regarding the crucial role played by FSE and inhomogeneity on the BKT transition in our Bi 2 Te 3 (7 QLs)/FeTe heterostructure as well as discuss the validity of our BKT analysis. First, in the infinite-size homogeneous case, the best fit using the infinite-size formula in ref. 32 (where and are the reduced temperatures) for the R – T data of our Bi 2 Te 3 (7 QLs)/FeTe sample is obtained with fitted parameters of b ~\n0.98, T BKT ~\n10.1 K and mean-field T c ~\n11.1 K. Thus the range between the mean-field T c and T BKT covers from 11.1 to 10.1 K, which is consistent with the temperature range used in the fittings presented in Fig. 4c,d . The value of the parameter ‘ b ’ in the equation of R ( T ) ∝ R 0 exp[− b /( T − T BKT ) 1/2 ] mentioned above is determined to be ~\n2.1 in fitting the standard BKT model. The fact that ‘ b ’ is in the order of 1, is consistent with the expectation of a recent theoretical model [33] . Here, ‘ b ’ was mentioned as a material parameter in the related works regarding 2D superconductors [3] , [6] . As pointed out in ref. 33 , ‘ b ’ appears in the exponential expression for the BKT correlation length . ‘ b ’ is meaningful in the sense that it appears in the condition for the use of the correlation length equation mentioned above. In our case, at the lower limit when , thus, well satisfies the condition. In addition, the rounding of the transition near R =0 in the R–T curve shown in Fig. 2a is expected to be due to FSE. Based on ref. 33 , we divided the R–T transition into four regions, GL-fluctuation region, BKT-transition region, FSE-dominated region and superconducting region, as shown in Fig. 5 , where the data are well fitted with the interpolating formula in ref. 33 for an inhomogeneity effect model (red curve). At T < T BKT , FSE arises and the normalized resistance starts to deviate from the infinite-size limit (black curve). As described in ref. 33 , inhomogeneity effects (or FSE) is associated with the scale of the sample dimensions or even smaller, and even though the system does not have a true granular structure, the homogeneous regions will have a typical size L hom smaller than the physical size L phys of the sample. The physical dimension of our sample is L phys ~\n500 μm and the critical current at T BKT is I c ~\n5 × 10 −3 A. Using the equation shown in ref. 33 , the characteristic length scale of our sample is estimated to be L hom ~\n0.3 μm. As expected by ref. 33 , L hom < L phys will give rise to a critical current for linear-to-nonlinear characteristic larger than expected for the homogeneous case, which is also consistent with the characteristics of j c versus T relationship of our sample as shown in the inset of Fig. 2b . In the infinite-size homogeneous case, a jump is expected from α =3 to α =1, however, for both our heterostructure sample and the LAO/STO interface superconductor [3] , the α value seems to show a smooth transition rather than a sudden sharp jump. As explained in ref. 33 , when taking the FSE into consideration, the change of α will be observed to possess a smooth downturn near T BKT , which is exactly what we observed in our data. 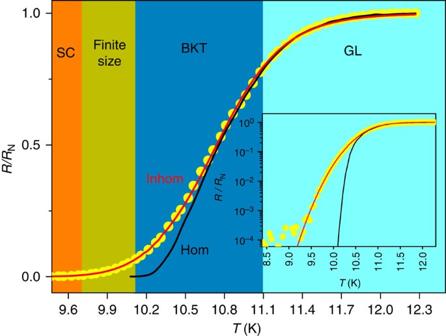Figure 5: Characteristic regions inR–Tcurve. The normalizedR–Tcurve of Sample A is plotted in four regions covering from GL, BKT, FSE to SC. The inset shows the same curve in a logarithmic plot. The red curve is a fit with the interpolating formula in ref.33for an inhomogeneity effect model, while the black curve is a fit based on the infinite-size limit. Figure 5: Characteristic regions in R–T curve. The normalized R–T curve of Sample A is plotted in four regions covering from GL, BKT, FSE to SC. The inset shows the same curve in a logarithmic plot. The red curve is a fit with the interpolating formula in ref. 33 for an inhomogeneity effect model, while the black curve is a fit based on the infinite-size limit. Full size image To reveal the origin of the 2D superconductivity at the interface of the heterostructure through either a theoretical or an experimental approach always remains to be a big challenge. Based on the data extracted from Fig. 2a , one can relate T c(onset) of the Bi 2 Te 3 /FeTe heterostructures with the Bi 2 Te 3 -thickness. As shown in Fig. 2c , T c(onset) increases steadily with the increase of the thickness of Bi 2 Te 3 , and then reaches a plateau value of ~\n11.5 K when the thickness of Bi 2 Te 3 reaches 5 QLs, a critical thickness that sets the length scale of Bi 2 Te 3 for observing the 2D superconductivity. Such dependence seems to suggest that chemical doping of FeTe, perhaps involving Bi, may be the cause of the observed superconductivity. This possible mechanism was investigated by carrying out atomic-resolution energy-dispersive X-ray spectroscopy (EDS) mapping across the Bi 2 Te 3 /FeTe interface as shown in Fig. 1d , which however shows that the fall of the Bi profile at the interface is quite sharp within the spatial resolution limit of atomic-resolution EDS derived from atomically sharp interfaces [34] . We have also performed extrinsic Bi doping of FeTe in two approaches, one with an elemental Bi source and the other with a Bi 2 Te 3 compound source (more details can be found in Supplementary Discussion ). It was found that the R versus T behaviours of these samples do not show any superconductivity feature. Both the results of atomic-resolution EDS and extrinsic Bi doping described above seem to imply that the observed 2D superconductivity at the Bi 2 Te 3 /FeTe interface may not be caused by Bi incorporation in the FeTe layer. We also provide a discussion about possible intrinsic Te doping in the FeTe layer in the Supplementary Discussion , which also implies that intrinsic Te doping is also unlikely to be the cause of the observed superconductivity. It is also worth to point out that one may argue this superconductivity may come from strain-induced superconductivity in FeTe as observed when FeTe was grown on lattice-mismatch substrates [35] . However, the growth of the top Bi 2 Te 3 layer on the bottom FeTe layer of the heterostructures studied in this work is via vdW epitaxy that is believed not to introduce substantial lattice distortion on both layer components. This is further confirmed by the results of a statistical approach used to determine the lattice parameters of FeTe and Bi 2 Te 3 . Figure 1e shows the variation of the lattice parameters of FeTe (left) and Bi 2 Te 3 (right) extracted from their HAADF images. As can be seen in this figure, except a small crystalline distortion appears in a portion of FeTe near the FeTe/ZnSe interface; the lattice parameters ( a and c ) of both the Bi 2 Te 3 and FeTe portions away from the Bi 2 Te 3 /FeTe interface well match with their bulk values. Thus, significant strain built up at the interface of the heterostructure is unlikely. As discussed above, the anomalous high j c and H C2 of the Bi 2 Te 3 /FeTe heterostructure sample are similar to those observed in Se doped FeTe thin films, in which the antiferromagnetic order of the parent FeTe is destroyed and the sample becomes superconducting. This indicates that the superconductivity of the Bi 2 Te 3 /FeTe heterostructure may be associated with the appearance of a superconducting layer of FeTe near the interface. It is possible that the significantly n-doped Bi 2 Te 3 thin film, with the presence of the topological surface states, may increase the electron density of the FeTe layers near the interface. This change of electron density may destroy the antiferromagnetic order of FeTe [22] and turn it into a superconductor. The Bi 2 Te 3 thin film fabricated in our molecular beam epitaxy (MBE) system has been previously characterized to be significantly n-doped with the Fermi level lying above the bottom of the conduction band [36] . As shown by Li et al . [37] , by performing angle-resolved photoemission spectroscopy on MBE-grown Bi 2 Te 3 thin films, the surface states can even be detected for thin films down to a single QL of Bi 2 Te 3 even though an energy gap opens near the Dirac point due to the coupling between the top and bottom surface states. Within this energy gap, the surface states do not exist as expected. However, the surface states still exist at a chemical potential well above the Dirac point, for example, when the sample is heavily n-doped. Therefore, observing reasonably strong superconductivity for heterostructures with Bi 2 Te 3 thin film down to a single QL does not rule out that surface states may play a role in the emergence of superconductivity in these samples. Moreover, the work of Li et al . [37] also reveals that as the thickness of Bi 2 Te 3 increases towards 5 QLs, the surface states reach their full topological nature, which means 5 QLs sets the length scale of fully-developed surface states for Bi 2 Te 3 . In our case, as shown in Fig. 2c , , 5 QLs is a critical thickness that sets the length scale of Bi 2 Te 3 for observing the 2D superconductivity. Since the two length scales mentioned above happen to coincide with each other, it may indicate that the topological nature of Bi 2 Te 3 and the observed 2D superconductivity perhaps are correlated with each other. However, it should be pointed out that as the Fermi level of our Bi 2 Te 3 layer lies above the bottom of the conduction band, the roles of the surface states and bulk states of Bi 2 Te 3 cannot be distinguished. Further studies, such as realizing an intrinsic Bi 2 Te 3 layer or tuning the Fermi level to coincide with the Dirac point through either extrinsic doping or adjusting gate bias, may help to clarify this issue. Below, the novelty and importance of this work are addressed. As compared with the superconductivities found in oxide heterostructures and arrays of superconducting islands on gold [38] , our work enjoys several novelties: first, an important novelty lies on the difference in the constituents of the materials. The interface superconductivity of our Bi 2 Te 3 /FeTe heterostructure likely requires the delicate interplay between the non-superconducting TI Bi 2 Te 3 and the non-superconducting parent compound of Fe-based superconductor FeTe. Our heterostructure system forms a novel platform for studying the interactions between these two new quantum states of matters. On the other hand, the superconductivity at the interface of oxide heterostructures (like LAO/STO) arises from the interplay of two traditional oxides. Moreover, the optimal T c of our system is about 12 K which is 50 times higher than the T c found in LAO/STO. Second, to the best of our knowledge, our Bi 2 Te 3 /FeTe heterostructure and the one unit-cell-thick FeSe grown on SrTiO 3 substrate [9] , [11] are the only 2D superconductivity systems, reported so far, that consist of an iron-chalcogenide component. The 2D superconductivity of our heterostructure distinguishes from that of the latter system by the fact that it arises from an addition of a new component (Bi 2 Te 3 ), while the latter simply relies on its own dimensionality reduction. Third, comparing with the other 2D superconducting systems reported so far, the Bi 2 Te 3 layer in our heterostructure enjoys a strong intrinsic spin-orbit coupling [20] while the inversion symmetry of the observed 2D superconductivity is broken at the interface, this combination could give rise to Rashba-type spin-orbit interactions and cause unconventional superconducting paring symmetry at the interface, similar to the LAO/STO system in which Rashba spin-orbit coupling is important for the formation of the helical Fulde–Ferrell–Larkin–Ovchinnikov states [39] . Fourth, our work provides the first example of interface superconductivity between a TI and iron chalcogenide. Due to the possible unconventional pairing symmetry of Fe-based superconductor [19] , the Bi 2 Te 3 /FeTe heterostructures also provide new platforms for creating and studying Majorana fermions in a 2D template, while several previous attempts have been made to induce superconductivity on TIs using bulk traditional superconductors. Film growth All the samples studied in this work were synthesized by a VG-V80H MBE system. Each sample contains a ZnSe buffer layer (50 nm) firstly deposited on the GaAs (001) semi-insulating substrates, followed by a deposition of FeTe with a thickness of 140 nm. The Bi 2 Te 3 /FeTe heterostructure samples were fabricated with varying thicknesses of the Bi 2 Te 3 thin films of 1, 2, 3, 5, 7, 9 and 14 QLs. A special heterostructure sample with Bi 2 Te 3 (7 QLs) deposited on only half of the FeTe (140 nm) surface was prepared by partially covering the FeTe surface with a tantalum strip in situ prior to the deposition of Bi 2 Te 3 . Device fabrications and transport measurements Each sample was cut into long strips using diamond scriber. Silver paint was used to form circular electrodes with diameters of ~\n0.5 mm and spacing of ~\n2.0 mm, which were connected to the measuring instruments with aluminium wires. Silver has long been characterized as a fast diffuser in Bi 2 Te 3 [40] , [41] . Based on our calculation using these findings in this reference, it takes the silver paint just 7 min to diffuse to a depth of 100 nm in Bi 2 Te 3 . Thus, it is likely that our silver paint electric contacts should penetrate the entire Bi 2 Te 3 thin film and reach the interface of the heterostructure and beyond. All the transport measurements were carried out in a Quantum Design PPMS system, which is equipped with a 14-T superconducting magnet and possesses a base temperature of 2 K. The transport measurements were conducted using a pulse mode to avoid heating effect, which was indeed found to be negligible for our measurements as consistent results were obtained when either the samples were placed in the Helium-4 vapour or in the Helium-4 liquid. For the heterostructure samples with thicknesses of 1, 2 and 3 QLs of Bi 2 Te 3 , the measuring temperature was further cooled down to 280 mK in an Oxford Cryostat with Helium-3 insert. How to cite this article : He, Q. L. et al . Two-dimensional superconductivity at the interface of a Bi 2 Te 3 /FeTe heterostructure. Nat. Commun. 5:4247 doi: 10.1038/ncomms5247 (2014).